Spin–orbit coupling in surface plasmon scattering by nanostructures The spin Hall effect leads to the separation of electrons with opposite spins in different directions perpendicular to the electric current flow because of interaction between spin and orbital angular momenta. Similarly, photons with opposite spins (different handedness of circular light polarization) may take different trajectories when interacting with metasurfaces that break spatial inversion symmetry or when the inversion symmetry is broken by the radiation of a dipole near an interface. Here we demonstrate a reciprocal effect of spin–orbit coupling when the direction of propagation of a surface plasmon wave, which intrinsically has unusual transverse spin, determines a scattering direction of spin-carrying photons. This spin–orbit coupling effect is an optical analogue of the spin injection in solid-state spintronic devices (inverse spin Hall effect) and may be important for optical information processing, quantum optical technology and topological surface metrology. Spin is an inherent universal property of any particle and characterizes an internal degree of freedom. The polarization state of light, being a classical electromagnetic notion, can be directly related to the quantum spin of a photon via the classical-quantum correspondence principle. Being fundamentally different from a statistical point of view, electrons (half-integer spin) and photons (integer spin) nevertheless exhibit several similar spin-related properties. One remarkable example is the spin Hall effect (SHE), originating from spin–orbit coupling. In the electronic SHE, electrons with opposite spins undertake different trajectories in a current flow [1] . In optics, photons with opposite spins—left or right circularly polarized (LCP or RCP) light—may propagate in different directions upon interaction with the material environment if spin–orbital coupling is engineered using, for example, metasurfaces [2] , [3] , [4] , Berry phase [5] , refractive index gradient [6] or near-field interference [7] . Here we describe and experimentally demonstrate the spin–orbit coupling effect manifested in the directional scattering of electromagnetic waves with opposite spins using the interaction of surface plasmon polariton (SPP) waves propagating on a metal interface with nanostructures. The effect is based on the reciprocity of optical interactions and the peculiar transverse angular momentum specific to surface electromagnetic waves on a metal–dielectric interface. While in the direct photonic SHE (PSHE), the polarization of the incident light controls the direction of the SPP excitation on a surface [2] , [3] , [4] , [5] , [6] , [7] , in the reciprocal scenario, in analogy to the spin injection current control in solid-state spintronic devices (inverse SHE) [8] , the direction of the scattered light of a given polarization is determined by the direction of the SPPs impinging at a scatterer. Model considerations In contrast to light beams that generally have both spin and orbital angular momenta oriented along the wavevector in free space, an SPP [9] , being a longitudinal wave with electric field components both parallel to the wavevector ( ) and perpendicular to the surface ( ; Fig. 1 ), has a purely transverse spin angular momentum oriented in the direction ( direction), perpendicular to the SPP wavevector [10] , [11] . This is a result of its elliptically polarized electric field in the k – z plane ( Fig. 1c ; Supplementary Note 1 ). This form of transverse angular momentum can also be observed in free space by engineering the optical field near a tight focal spot [12] . SPP fields, being transverse-magnetic in nature, have a mirror symmetry in the k – z plane. The fields scattered by any mirror-symmetric structure will therefore satisfy the same symmetry. As a consequence, any RCP field produced by SPPs scattered at any given angle is mirrored with a LCP field radiated in the mirror-symmetric direction ( Supplementary Note 1 ). The spin of both scattered fields will add up to a positive non-zero spin along the ( x direction). If the propagation direction of the SPP is reversed, so will the spin of the scattered photons, forming the basis of the inverse PSHE. 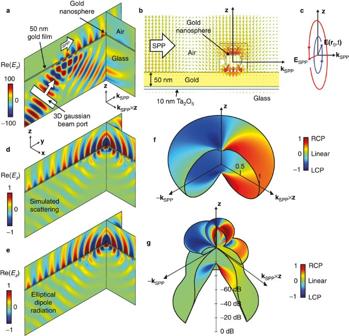Figure 1: Concept of spin–orbit coupling in SPP scattering by a spherical nanoparticle. (a) SimulatedEzfield of the Gaussian beam exciting SPPs that propagate towards the nanosphere. (b) Electric field structure (in they–zplane) of the SPP polarizing the sphere (snapshot fromSupplementary Movie 1). (c) Schematics of the electric field configuration inside the metal sphere,E(r0,t), and of the SPP,ESPP(r0,t), at the location of the sphere. (d) Scattering field distribution from the sphere obtained from the simulations by subtracting the background field. (e) Radiation field distribution of an elliptically polarized dipole (mimicking the scattering) placed atr0. (f) Far-field radiation pattern in free space (no substrate) for the elliptical dipole calculated using equation (1): the radius is the amplitude of the radiated field in linear scale, the colour scale is the Stokes parameter (|ERCP|2−|ELCP|2)/|E|2indicating the ellipticity of the radiation. (g) Numerically simulated far-field pattern (the radius is the amplitude in dB scale) for the elliptical dipole placed above the metal film and substrate. Figure 1: Concept of spin–orbit coupling in SPP scattering by a spherical nanoparticle. ( a ) Simulated E z field of the Gaussian beam exciting SPPs that propagate towards the nanosphere. ( b ) Electric field structure (in the y – z plane) of the SPP polarizing the sphere (snapshot from Supplementary Movie 1 ). ( c ) Schematics of the electric field configuration inside the metal sphere, E( r 0 ,t) , and of the SPP, E SPP ( r 0 ,t ), at the location of the sphere. ( d ) Scattering field distribution from the sphere obtained from the simulations by subtracting the background field. ( e ) Radiation field distribution of an elliptically polarized dipole (mimicking the scattering) placed at r 0 . ( f ) Far-field radiation pattern in free space (no substrate) for the elliptical dipole calculated using equation (1): the radius is the amplitude of the radiated field in linear scale, the colour scale is the Stokes parameter (| E RCP | 2 −| E LCP | 2 )/| E | 2 indicating the ellipticity of the radiation. ( g ) Numerically simulated far-field pattern (the radius is the amplitude in dB scale) for the elliptical dipole placed above the metal film and substrate. Full size image Simulations When the SPP wave impinges on a nanoparticle, the latter will become polarized ( Fig. 1b , Supplementary Movie 1 ). Assuming an isotropic polarizability α for the nanoparticle, the SPP-induced dipole p is related to the impinging spin-carrying SPP fields as p = α E SPP ( r 0 ) and, therefore, describes an ellipse in the k – z plane ( Fig. 1c ), such as the dipole components satisfy where n SPP is the effective mode index of the SPP. When n SPP >>1, as is the case for an SPP near the surface plasmon frequency, the induced dipole polarization would be purely circular. For the experimental geometry and wavelength, n SPP ≈1.05+0.0007i, and, thus, radiation of the induced dipole p , will be elliptically polarized with a spin in the direction. As a result, the scattered light will have opposite handedness in mirror directions of the plane of symmetry. The assumption of an isotropic polarizability used in equation (1) is not exact for consideration of anisotropic objects, such as a slit or grating in a metal film; however, it is a good approximation as deduced by the similarity between the incident field E and the polarization p in simulations ( Fig. 1c ). Anisotropy is straightforward to include in the model and would not significantly alter the physics considerations behind the phenomenon. Figure 1d shows the full vectorial numerical modelling of the effect. A Gaussian beam illuminates a gold film from a glass substrate, exciting an SPP at the metal–air interface, which in turn impinges on a 60-nm-diameter gold nanosphere placed on the Au film. The scattered field distribution obtained numerically ( Fig. 1d ) is the same as analytically simulated for an induced dipole polarized according to equation (1) ( Fig. 1e ), confirming the model discussed above. Figure 1f shows the analytically calculated angular distribution of the scattered intensity of the dipole when placed in free space. Elliptically polarized radiation of opposite handedness is observed in opposite directions. The presence of the metal film and the substrate modifies the polarization distribution of the scattered field ( Fig. 1g ). While the intensity distribution is more complex, the same symmetry in photon spin distribution is maintained, confirming the general principle of the inverse effect. The polarization of scattered light follows a mirror symmetry with respect to a plane perpendicular to the spin of the incoming illumination. In this case, the incident SPP carries a transverse spin parallel to the surface of the metal ( x direction) and, therefore, x =0 is the mirror plane of the scattering. Experimental results In order to experimentally demonstrate the effect, we have characterized the SPP scattering from several nanostructures, including a nanoparticle, a nanoslit and a collection of slits forming a diffraction grating. As a starting point, Fig. 2a shows the direct PSHE [7] , [13] , where the scattering of circularly polarized light by a spherical metal nanoparticle leads to the directional excitation of SPP waves dependent on the wavevector and spin of incoming photons. SPPs are excited on a smooth metal film on the left or the right from the nanoparticle corresponding to the right-handed or left-handed polarization state of the illuminating light, respectively ( Fig. 2b,e and Supplementary Movie 2 ). By spatial filtering of the collected light in a Fourier plane of the imaging system, the leakage radiation from SPPs can be observed directly and the predicted dependence of the SPP directionality on the particular polarization state of the incident light observed. The maximum intensity ratio found to exceed 7:1 between the left- and right excited SPPs ( Fig. 2b ). For linearly polarized photons, corresponding to the superposition of LCP and RCP polarizations, no directionality is expected and a symmetric excitation of SPPs in both directions takes place. 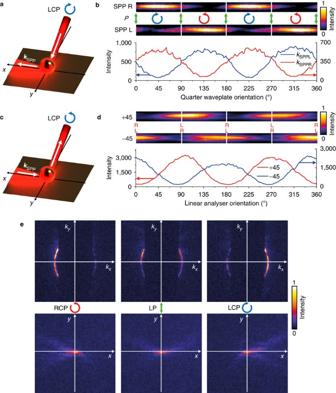Figure 2: PSHE and SPP scattering by a spherical nanoparticle. (a) Schematic of the direct PSHE experiment. (b) The intensity of the SPPs excited in opposite directions for a full set of incident polarization states from RCP through linear p-polarized to LCP. (c) Schematic of the reciprocal experiment. (d) The dependence of the intensity of the directionally scattered light on the polarizer orientation for two orthogonal quarter-waveplate orientations (marked as ‘+45’ and ‘–45’). For all measurements, the 60-nm-diameter Au nanoparticle is placed on the 50-nm-Au film on glass substrate. The illumination light wavelength is 632.8 nm. (e) The wavevector spectrum (top row) and corresponding real space intensity distribution (bottom row) of the SPP waves excited with LCP, linear p-polarized and RCP illuminating light (the snapshots fromSupplementary Movie 2). Figure 2: PSHE and SPP scattering by a spherical nanoparticle. ( a ) Schematic of the direct PSHE experiment. ( b ) The intensity of the SPPs excited in opposite directions for a full set of incident polarization states from RCP through linear p-polarized to LCP. ( c ) Schematic of the reciprocal experiment. ( d ) The dependence of the intensity of the directionally scattered light on the polarizer orientation for two orthogonal quarter-waveplate orientations (marked as ‘+45’ and ‘–45’). For all measurements, the 60-nm-diameter Au nanoparticle is placed on the 50-nm-Au film on glass substrate. The illumination light wavelength is 632.8 nm. ( e ) The wavevector spectrum (top row) and corresponding real space intensity distribution (bottom row) of the SPP waves excited with LCP, linear p-polarized and RCP illuminating light (the snapshots from Supplementary Movie 2 ). Full size image To observe the inverse effect, the nanoparticle on a metal surface is illuminated under reciprocal condition, that is, by SPP waves ( Fig. 2c ). Experimentally, the direction of the incident SPP can be controlled by focusing light in the back focal plane of the illuminating microscope objective and, thus, selecting the appropriate excitation light wavevector for coupling to the SPP propagating in a chosen direction. In this way, the inverse (SPP-to-light scattering) conditions for the previous (light-to-SPP scattering) measurements can be achieved (see Methods). As the SPP is scattered by the nanoparticle in the far field, the polarization analysis shows that the scattered light carries a net spin. The polarization state of scattered light in the direction outside the plane of incidence ( k – z plane) can be determined, including its handedness, by analysing it with a linear polarization filter placed after a quarter-wave plate. Although the scattering from the particle occurs in all directions, our experimental analysis of the polarization is limited to a single direction for simplicity ( Fig. 2c ). It can be seen that the scattered light is circularly polarized by noticing that it becomes almost linearly polarized at 90° and 0° for the quarter-wave plate orientations at +45° and −45°, respectively ( Fig. 2b ). This corresponds to left-handed elliptical polarization, in agreement with the handedness predicted by the theoretical considerations above. Using different types of scatterers, the role of spin–orbit coupling in the SPP scattering in circular-polarized light has been further confirmed ( Fig. 3 ). The effect is observed upon scattering of an obliquely incident SPP wave by both a slit and a collection of slits forming a diffraction grating. Here the scattered light exists at a particular k y equal to that of the incident SPP wave because of the nature of scattering from two-dimensional (2D) diffracting elements, invariant along one direction, in contrast to the previously examined three-dimensional nanoparticle. In this case it is easier (compared with a spherical nanoparticle) to analyse all possible scattering directions at different k x values, corresponding to different scattering angles. It is observed that for both the slit and grating, the scattered light at k x =0 has an almost constant intensity for all linear analyser orientations, indicating that it is close to circularly polarized ( Fig. 3b , top). The grating acts to further direct light in the selected spatial frequencies corresponding to the diffraction orders of the grating, preserving the properties of polarization of the scattered light from one slit described above ( Fig. 3b , bottom). In both cases, the light scattered at higher values of k x becomes increasingly linearly polarized. The polarization was not found to be fully circular in accordance with the theoretical modelling and experimental observation of direct PSHE on these nanostructures [7] . The direction of the scattered light with a given elliptical polarization and the polarization of the scattering light in the same direction can be simply controlled by changing the SPP propagation direction. 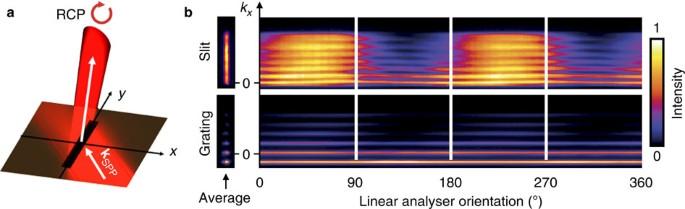Figure 3: SPP scattering by slits in a metal film. (a) Schematic of the SPP scattering measurements on a slit and a slit grating. (b) The dependence of the intensity of the scattered light on linear analyser orientation for the individual single slit with width 130 nm and length 20 μm (top), and diffraction grating consisting of a 1D array of slits with a slit width, length and periodicity of 500 nm, and 20 and 3 μm, respectively (bottom). The slits have been fabricated in a 50-nm-gold thin film. The observed diffraction pattern averaged over all analyser angles is shown on the left. Figure 3: SPP scattering by slits in a metal film. ( a ) Schematic of the SPP scattering measurements on a slit and a slit grating. ( b ) The dependence of the intensity of the scattered light on linear analyser orientation for the individual single slit with width 130 nm and length 20 μm (top), and diffraction grating consisting of a 1D array of slits with a slit width, length and periodicity of 500 nm, and 20 and 3 μm, respectively (bottom). The slits have been fabricated in a 50-nm-gold thin film. The observed diffraction pattern averaged over all analyser angles is shown on the left. Full size image The specific transverse spin topology, with the spin vector normal to the wavevector, is required to achieve opposite handedness in the opposite, mirror-symmetric scattering directions. Such transverse spin can be realized with an SPP wave, or other guided modes, or indeed in free space in special cases of light focusing [12] . The effect does not exist (for an isotropic particle) if the illuminating field does not possess such a spin structure. The induced polarization of the isotropic particle must follow the same polarization pattern as that of the incident light electric field. Therefore, the radiation of the induced dipole determining the particle scattering in free space in a given direction will only be circular or elliptical if the projection of the polarization ellipse in the plane perpendicular to the given direction is elliptical or circular. This translates into the requirement for the incident electric field to have a non-zero component of spin in that direction. In the case of an incident linearly polarized plane wave with no net spin, the isotropic particle becomes linearly polarized and radiates in a doughnut-shaped radiation diagram, but with linear polarization in all directions ( Fig. 4a ). If the incident circularly polarized plane wave has a spin in, for example, the + y direction (RCP-polarized light), the particle gets polarized circularly and radiates circular polarized light in the forward and backward directions ( Fig. 4b ). However, in any direction contained within the x – z plane (orthogonal to the incident light spin), the radiation is always linearly polarized because the projection of the particle polarization in a plane perpendicular to any direction in the x – z plane is always linearly polarized. An SPP-like field having longitudinal ( y direction) and transverse ( z direction) components while propagating in free space, with its spin transverse to the propagation ( y ) direction can be obtained in specifically focused beams [12] . In such a field, the particle will be polarized elliptically in the y – z plane ( Fig. 4c ), and then scatters light with elliptical polarizations mainly in the + x and − x directions, but with a symmetry plane perpendicular to the spin of the incident wave. This is the case similar to the one described above with SPPs. As long as an isotropic particle is considered, the scattered radiation can only have an elliptical or circular polarization in the directions in which the incident wave has the spin projection. In addition, symmetry considerations require that opposite handedness will be radiated in mirror-symmetric directions with respect to a mirror plane defined as normal to the initial spin of the incident electric field. This is in accordance with the conservation of angular momentum: the scattered field of a free standing particle (with rotational symmetry) will show the same angular momentum as the incident field. This will be an approximation when the particle is placed near a surface that breaks rotational symmetry. Thus, the transverse spin of the SPP is important for achieving opposite handedness in left and right mirror-symmetric directions. 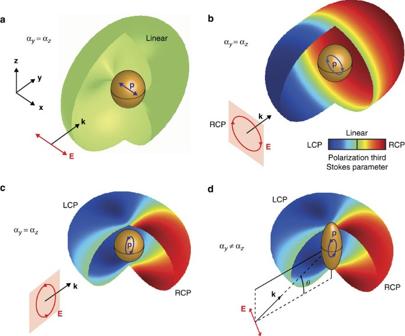Figure 4: Spin topology determines scattering polarization. Polarization of the scattered light by an isotropic polarizable particle in free space illuminated by light which is (a) linearly polarized, (b) circularly polarized with longitudinal spin and (c) circularly polarized with transverse spin. (d) Polarization of scattered light by an anisotropic particle illuminated by a linearly polarized plane wave at a tilted angleθ. Black arrow, incident light wavevector; red curve, trajectory followed by the electric field of the incident light; Blue curve, trajectory of the polarization of the particle that, for an isotropic particle, has the same shape as the incident electric field. Figure 4: Spin topology determines scattering polarization. Polarization of the scattered light by an isotropic polarizable particle in free space illuminated by light which is ( a ) linearly polarized, ( b ) circularly polarized with longitudinal spin and ( c ) circularly polarized with transverse spin. ( d ) Polarization of scattered light by an anisotropic particle illuminated by a linearly polarized plane wave at a tilted angle θ . Black arrow, incident light wavevector; red curve, trajectory followed by the electric field of the incident light; Blue curve, trajectory of the polarization of the particle that, for an isotropic particle, has the same shape as the incident electric field. Full size image Interestingly, with an anisotropic particle under a tilted illumination with a linearly polarized plane wave ( Fig. 4d ), it is possible to achieve a similar scattering behaviour without requiring the transverse spin topology of the incident light. The polarization of the particle in this case can be written as , where E 0 is the incident electric field amplitude, α i is the polarizability in the i = x , y , z directions and θ is the angle between the wavevector of the incident light and the y axis. In this case, the ratio of polarizabilities in equation (1) becomes where k z and k y are the wavevector components of the incident wave. To achieve circular polarizations radiated laterally, p y / p z should be a non-zero complex quantity (a real-valued ratio would lead to linear polarization). For plane wave illumination with a conventional longitudinal spin topology, this condition is possible to satisfy as long as θ ≠0 (tilted incidence, breaking the z -mirror symmetry of the system) and α y ≠ α z (anisotropic particle) with the ratio α y / α z being complex [14] . In the case of an anisotropic scatterer illuminated by a SPP wave, equation (1) leads to which is the mathematical generalization of equation (2) when applied to evanescent waves with a transverse spin, for which | k y |> k 0 and θ is imaginary. This condition implies an imaginary value for , and therefore achieves a complex value for the ratio p y / p z in equation (2), even if the particle is isotropic or α y / α z is real. Note that the required condition k y > k 0 is valid for any bound electromagnetic mode and is associated with the existence of a transverse spin corresponding to the evanescent electric field above a waveguiding structure (for example, fibre, planar waveguide or plasmonic interface) responsible for breaking the z -mirror symmetry of the isotropic particle/waveguide system. The consideration of polarization degree of freedom in electromagnetic waves paves the way for a variety of novel optical effects, like optomechanical forces [15] and mimicking spintronics [16] and spin-based electronic circuits [17] , where additional (spinor) degree of freedom extends the space of scalar wavefunctions to vectorial variables. An optical analogue of the inverse SHE described here in scattering of highly confined plasmonic waves on metal–dielectric interface, capable of carrying transverse spin, may ultimately serve as the platform for conventional or quantum electromagnetic signal processing, providing, among others, an integrated source of LCP/RCP-entangled photons [18] , [19] , orbital angular momentum entanglement [20] , [21] and platforms for testing fundamental laws of nature [22] . Being a fundamental optical effect, it also brings cross-disciplinary similarities, for example, spin–current injections and related effects in solid-state electronic devices. Control of the state of light polarization in such an integratable manner also puts on the agenda spintronic–spinoptical integrated circuitry, enabling the control of individual electron spins in semiconductor structures [23] . With reciprocal control of emission/absorption in spin-selective quantum dots and waveguided mode excitation control, other applications may exist in quantum information processing with efficient in/out coupling to spin-sensitive quantum emitters of single photons. Samples The 60-nm-spherical nanoparticles studied in this work ( Supplementary Fig. 1 ) were deposited on a 50-nm-gold thin film by a drop cast method from a colloidal solution of monodisperse Au nanoparticles (BBinternational). The film itself was fabricated by magnetron sputtering on a glass cover slip with a 10-nm layer of Ta 2 O 5 for adhesion purposes. The slit structures studied in this work ( Supplementary Fig. 1 ) were directly patterned by the focussed ion beam milling of the same 50-nm-Au thin film. The individual slit width and length were 130 nm and 20 μm, respectively. The grating (a one-dimensional (1D) array of slits with a slit width, length and periodicity of 500 nm, and 20 and 3 μm, respectively) was fabricated in a similar manner as the individual slit. Optical measurements The optical set-up for the observations of the direct and inverse PSHEs is shown in Supplementary Fig. 2 . For PSHE studies, coherent light from a He–Ne laser at a wavelength of 632.8 nm was passed through a linear polarizer and a λ /4 plate and then directed towards the nanoparticle or collinearly with the slit structures at an incident angle of 70° with respect to the metal surface. The sample was mounted on an inverted microscope and light scattered in the glass substrate was collected using a high numerical aperture oil immersion objective (1.49). The resulting real space image of the scatterer was spatially filtered in order to only detect light from the smooth metal surface in the vicinity immediately next to the scatterer and, thus, avoid the collection of directly scattered light from the structure. This filtered image was then mapped into Fourier space (spatial frequency spectrum) by means of an optical Fourier transform using a series of lenses. The direct zero-order transmission through the film was blocked by another spatial filter and the remaining light was re-imaged as either a real or reciprocal space image on to an intensified CCD array. For the reciprocal space image, the recorded intensity distribution corresponds directly to the angular distribution of the light collected from the spatially filtered region. The leakage radiation collected from SPPs excited on the metal–air interface by the scattering structures in this configuration may, depending on the scattering from the structure, appear anywhere on the SPP cone slightly beyond the light cone of air; however, the wavevectors will be concentrated around the same k y as the incident radiation. For the real space image, the intensity distribution is in this case, a spatial map directly showing propagating SPPs leaking through the film and into the substrate. For the reciprocal measurements ( Supplementary Fig. 2b ), coherent light from a He-Ne laser at a wavelength of 632.8 nm was spatially filtered and the beam was expanded before passing through a linear polarizer. This collimated beam was then focussed to a diffraction-limited point in the Fourier space that corresponds to the particular in-plane scattering angle, that is, wavevector, for the excitation of an SPP propagating on the Au–air interface in a chosen direction (the incident linear polarization is then tuned appropriately). The SPP is thus directed in this manner to impinge upon a scatterer on the substrate. The wavefront scattered back through the film is then passed through the collection system as in Supplementary Fig. 2a . In this case, an aperture is used as a spatial filter in a real space image plane in order to select the area immediately around the particle and thus block the majority of zero-order scattering. A second aperture is placed appropriately in the Fourier plane in order to further reject this unwanted light. The light is then passed through the polarization analysing elements placed in a quasi-collimated plane before being projected on to the intensified CCD array as either a real or reciprocal space image. Modelling Analytical model of the transverse spin–orbit coupling is described in Supplementary Note 1 . The numerical simulations were carried out using the CST Microwave Studio’s time-domain finite-element method. A Gaussian beam was directed at the metal plane from the substrate in order to excite SPPs on the metal–air interface. The SPPs propagate along the top interface of the metal film and reach the spherical particle. The simulation had open boundaries in all directions. The scattering from the nanoparticle is obtained by subtracting, in MATLAB, the total fields, from the incident fields, obtained by simulating the same structure without the scatterer. The polarization of this scattered light was then analysed. The material properties were modelled at the wavelength of 632.8 nm as follows: the glass substrate was considered with a refractive index n glass =1.45, the 10-nm sticking Ta 2 O 5 layer with n s =1.80 and the 50-nm gold layer with ε Au =−11.8+1.239 i (CST dispersive model fit). The simulated mesh had a cell size of λ /15, locally improved to 10 nm in the metal and to 5 nm inside and in the vicinity of the scattering sphere of 60 nm diameter. How to cite this article: O’Connor, D. et al. Spin–orbit coupling in surface plasmon scattering by nanostructures. Nat. Commun. 5:5327 doi: 10.1038/ncomms6327 (2014).